Site-specific cleavage of bacterial MucD by secreted proteases mediates antibacterial resistance inArabidopsis Plant innate immunity restricts growth of bacterial pathogens that threaten global food security. However, the mechanisms by which plant immunity suppresses bacterial growth remain enigmatic. Here we show that Arabidopsis thaliana secreted aspartic protease 1 and 2 (SAP1 and SAP2) cleave the evolutionarily conserved bacterial protein MucD to redundantly inhibit the growth of the bacterial pathogen Pseudomonas syringae . Antibacterial activity of SAP1 requires its protease activity in planta and in vitro. Plants overexpressing SAP1 exhibit enhanced MucD cleavage and resistance but incur no penalties in growth and reproduction, while sap1 sap2 double mutant plants exhibit compromised MucD cleavage and resistance against P. syringae . P. syringae lacking mucD shows compromised growth in planta and in vitro. Notably, growth of ΔmucD complemented with the non-cleavable MucD F106Y is not affected by SAP activity in planta and in vitro. Our findings identify the genetic factors and biochemical process underlying an antibacterial mechanism in plants. During the course of co-evolution with microbial pathogens, plants and animals have evolved highly sophisticated innate immune systems to defend themselves against pathogen infection [1] , [2] . In both systems, specific host receptors recognize microbial molecules, thereby activating cellular signaling pathways that eventually contribute to the suppression of pathogen growth [3] , [4] , [5] . The immune system needs to be tightly controlled because over activation causes autoimmune diseases in humans and often involves growth retardation in plants. This so-called immunity-growth tradeoff in plants poses a dilemma in agriculture [6] , [7] , [8] . Activation of host immune signaling pathways leads to the production of antimicrobial molecules and cellular changes in the host that directly alters microbial metabolisms, resulting either in pathogen growth suppression or demise [2] , [9] . In animals, circulating immune cells exert antibacterial activity through multiple extensively studied mechanisms [10] , [11] , such as direct bacterial killing, activation of antimicrobial peptides, and attenuation of bacterial virulence by secreted proteases [12] , [13] . On the other hand, evidence for how plants suppress bacterial growth is rather limited. Plants produce antimicrobial peptides or secondary metabolites, which have antibacterial properties in vitro, but their physiological relevance and modes of action in plants remain obscure [14] . Many plant proteases are predicted to be secreted into the extracellular space (apoplast), which is an important niche for leaf bacterial pathogens [15] , [16] , [17] , [18] , [19] . Some secreted proteases play roles in plant immunity. For instance, the extracellular subtilase SBT3.3 positively contributes to resistance against bacterial and fungal pathogens in Arabidopsis thaliana as the absence or overexpression of SBT3.3 leads to susceptibility or resistance, respectively [17] . Similarly, a secreted aspartic protease CDR1 is an important player during immunity against bacterial pathogens in A. thaliana as well as in rice [20] , [21] . Pip1 is a secreted papain-like protease that contributes to resistance in tomato against pathogens across multiple kingdoms [19] . Plant pathogens produce protease inhibitors to counteract the host proteases, supporting the idea that plants and pathogens engage in protease warfare on the battleground in the apoplast [22] . Although the studies above have provided strong evidence that secreted proteases are important components of plant immunity, both SBT3.3 and CDR1 carry out their roles by activating plant immune signaling pathways [17] , [21] , and their target for immunity remains unknown [22] . In the present study, we provide compelling biochemical and genetic evidence that A. thaliana secretes the secreted aspartic protease 1 (SAP1) and SAP2 to cleave the bacterial protein MucD, thereby suppressing Pseudomonas syringae growth in the leaf apoplast. Both SAP and mucD are evolutionarily conserved in the plant and bacterial kingdoms, respectively. Our work, therefore, sheds light on the previously poorly understood mechanisms by which plants protect themselves against bacterial pathogens. SAP1 and SAP2 suppress P. syringae growth in planta Foliar bacterial pathogens colonize the extracellular space, and thus to gain insights into how plant immunity suppresses bacterial growth in the leaf apoplast, we tested the ability of immune-activated apoplastic fluid (from leaves treated with the flg22 peptide from bacterial flagellin) to suppress bacterial growth in vitro. This apoplastic fluid suppressed growth of P. syringae pv. tomato DC3000 ( Pto ) compared to that from water-treated leaves, and this effect was heat sensitive (Fig. 1a ), implying that a protein is responsible. We reasoned that secreted proteases are plausible candidates as they would be able to directly target bacterial protein in the apoplast. The A. thaliana genome contains over 700 genes encoding putative proteases [23] . We focused on aspartic proteases as they generally have optimum activity at the acidic pH of the plant apoplast [24] , [25] , [26] . We found 77 A. thaliana aspartic proteases in MEROPS [27] (Supplementary Fig. 1A ). Sixty-one possess an N-terminal secretion signal peptide [28] , and 51 are predicted to have extracellular localization in TAIR10 [29] . Of these, two tandemly arrayed genes ( At1g03230 and At1g03220 ), whose expression was not distinguishable by microarray-based system due to their high sequence similarity in Genevestigator, show consistent induction by both flg22 and Pto [30] (Supplementary Fig. 1A ). Since these genes have not been previously described, we termed them SAP1 and SAP2 , respectively. Fig. 1 Secreted aspartic protease 1 (SAP1) and SAP2 are induced and secreted during P. syringae infection. a In vitro growth of Pto (OD 600 = 0.05) amended with apoplastic fluid from leaves of -week-old Col plants at 24 h post infiltration (hpi) with 1 µM flg22 or mock or boiled apoplastic fluid (boiled) was measured at 9 h after culturing. Bars represent means and s.e.m. of three independent experiments each with eight replicates. Statistically significant differences are indicated by different letters (adjusted P < 0.05). b Expression of SAP1 and SAP2 in leaves of 4-week-old Col plants at 1 or 24 hpi with mock, 1 µM flg22, or Pto (OD 600 = 0.001). Bars represent means and s.e.m. of three biological replicates. Asterisks indicate significant differences (Student’s two-tailed t test; * P < 0.05, ** P < 0.01). c Accumulation of SAP1-GFP (green fluorescent protein) and SAP2-GFP at 1 day post infiltration (dpi) with Pto (OD 600 = 0.001) or mock determined by immunoblotting using an anti-GFP antibody. Rubisco large subunit (RbCL) and PR1 serve as controls for total and apoplastic proteins, respectively. d SAP1-RFP (red fluorescent protein) and SAP2-RFP (red color) with or without the signal peptide (ΔSP) were expressed from the 35S promoter by Agrobacterium -mediated transient transformation in transgenic A. thaliana plants expressing plasma-membrane-localized WAVE131-YFP (yellow fluorescent protein) (green color). YFP and RFP fluorescence signals were detected at 2 dpi. The intensity of YFP and RFP fluorescence signals was quantified along the dotted lines using ImageJ software (left to right). Four independent experiments were performed with similar results Full size image We determined the individual expression levels of SAP1 and SAP2 by quantitative reverse transcription PCR (RT-qPCR). Both SAP1 and SAP2 expression was induced upon flg22 treatment and Pto infection (Fig. 1b ). Immunoblotting of the SAP fusion proteins showed slightly increased apoplastic accumulation upon Pto infection (Fig. 1c ). To test if the apoplastic localization was signal peptide dependent, full-length SAP1-RFP or SAP2-RFP or signal peptide-depleted SAP1 (ΔSP)-RFP or SAP2 (ΔSP)-RFP , driven by a constitutive ubiquitin promoter, were transiently expressed in A. thaliana transgenic plants expressing a plasma-membrane-localized GFP (green fluorescent protein) (WAVE131) [31] . RFP (red fluorescent protein) signals were detected between GFP signals in a signal-peptide-dependent manner (Fig. 1d ), suggesting that SAP1 and SAP2 are secreted into the apoplast via the canonical protein secretion pathway [32] , [33] . Two independent T-DNA insertion mutants for SAP1 , SALK_062079 ( sap1-1 ) and SAIL_646_E08 ( sap1-2 ), were obtained, and disruption of SAP1 was confirmed in both lines (Supplementary Fig. 1B, C ). We also generated SAP2 RNA interference (RNAi) and CRISPR-Cas9-knockout lines in wild-type Col as well as in sap1-1 background since no sap2 T-DNA insertion lines were available (Supplementary Fig. 1D, E ). Only sap1 sap2 CRISPR-Cas9 knockout ( sap1 sap2 ) and sap1 SAP2 -RNAi plants exhibited increased susceptibility to Pto , while single mutant and SAP2 -RNAi plants did not, implicating that SAP1 and SAP2 redundantly contribute to resistance against Pto (Fig. 2a and Supplementary Fig. 1F ). We also generated transgenic A. thaliana plants, which constitutively express either the full-length SAP1 or SAP2 or SAP1ΔSP or SAP2ΔSP , all of which were generated as fusion proteins with RFP at the C terminus. We observed decreased bacterial growth in transgenic plants expressing the full-length SAP1-RFP or SAP2-RFP as compared with wild-type Col plants but not in plants expressing SAP1ΔSP or SAP2ΔSP , which localized to the cytosol (Figs. 1d , 2b ). Immunoblotting confirmed that protein expression levels were comparable in all transgenic lines (Fig. 2b ). Thus, the apoplastic localization of SAP1 and SAP2 is essential for bacterial growth suppression. Enhanced disease resistance is often associated with constitutive immune activation and a consequent growth penalty [6] , [7] , [8] . Interestingly, none of transgenic plants showed enhanced expression of the immune marker PR1 , except for pUB::SAP2 line 2 with a slight increase, growth retardation, or reduced reproduction, but some of them showed enhanced growth and reproduction (Fig. 2c–f ). These data imply that SAP1 and SAP2 influence bacterial proliferation via direct interaction with bacteria in the apoplast, and that their overexpression poses minimal plant fitness costs. Fig. 2 Secreted aspartic protease 1 ( SAP1 ) and SAP2 redundantly contribute to resistance against P. syringae . a Leaves of 4-week-old Col, sap1 , sap2 , and sap1 sap2 double mutant plants were infiltrated with Pto (OD 600 = 0.0005), and bacterial titer was determined at 3 days post infection (dpi). Bars represent means and s.e.m. of four independent experiments with three biological replicates. Asterisks indicate significant differences from Col (Student’s two-tailed t test; * P < 0.05, ** P < 0.01). b Leaves of 4-week-old pUB::SAP1-RFP (red fluorescent protein) and SAP2-RFP with or without signal peptide ( ΔSP ) were infiltrated with Pto (OD 600 = 0.001), and bacterial titer was measured at 2 dpi. Bars represent means and s.e.m. of three independent experiments with at least three biological replicates. Asterisks indicate significant differences from Col (Student’s two-tailed t test; * P < 0.05, ** P < 0.01). Protein expression determined by immunoblotting using an anti-RFP antibody. Ponceau S staining serves as protein loading control. c , i Relative expression of PR1 in leaves of 4-week-old Col, pUB::SAP1-RFP , pUB::SAP1ΔSP-RFP , pUB::SAP2-RFP , pUB::SAP2ΔSP-RFP , and pUB::SAP1 D63/136A plants were determined by quantitative reverse transcription PCR (RT-qPCR). Bars represent means and s.e.m of three biological replicates. The vertical axis shows the log 2 expression levels relative to Actin2 . Col plants 24 h post infiltration (hpi) with flg22 serves as a positive control for activated PR1 expression. Asterisks indicate significant differences from Col (Student’s two-tailed t test; * P < 0.05, ** P < 0.01). d , j Phenotype of 4-week-old leaves of Col, pUB::SAP1-RFP and pUB::SAP2-RFP , and pUB::SAP1 D63/136A plants. Shoot fresh weight (4-week-old; e ) and silique numbers ( f ) of Col, pUB::SAP1-RFP , pUB::SAP1ΔSP-RFP , pUB::SAP1 D63/136A -RFP, pUB::SAP2-RFP , and pUB::SAP2ΔSP-RFP plants. Bars represent means and s.e.m. of three independent experiments each with four biological replicates ( e ) or means and s.e.m. of three independent experiments ( f ). Statistically significant differences are indicated by different letters (adjusted P < 0.01). g Protein expression of SAP1 and SAP1 D63/136A in Col, pUB::SAP1-RFP and pUB::SAP1 D63/136A -RFP plants by immunoblotting using an anti-RFP antibody. Rubisco large subunit (RbCL) serves as a loading control. Three independent experiments were performed with similar results. h Leaves of 4-week-old Col and pUB :: SAP1 D63/136A plants were infiltrated with Pto (OD 600 = 0.001), and bacterial titer was measured at 2 dpi. Bars represent means and s.e.m, of four independent experiments with four biological replicates. n.s., not significant Full size image SAP1 and SAP2 suppress P. syringae growth in vitro To test if SAP1 and SAP2 suppress bacterial growth by direct interaction, we produced in Escherichia coli and purified recombinant SAP1ΔSP and SAP2ΔSP fused to GST at the C terminus. As compared with the GFP control, both SAP1 and SAP2 showed protease activity, which was blocked by an aspartic protease inhibitor, pepstatin A (Fig. 3a ). These active SAP1 and SAP2 proteins, but not the heat-inactivated or GFP controls, suppressed in vitro Pto growth (Fig. 3b ). In MEROPS, SAP1 and SAP2 are classified into Clan AA Family A1, which includes an A. thaliana aspartic protease involved in immune activation, CDR1 [21] , [34] . Aspartic proteases generally require two conserved Asp residues that intramolecularly form the catalytically active site, although some are known to form a homodimer that intermolecularly generates an active site consisting of two Asp residues [35] . SAP1 and SAP2 are described as “non-peptidase homologs,” as they lack one of the Asp residues in the active site. Sequence alignment revealed that one of the catalytically essential Asp residues in CDR1 is replaced with Ser in SAP1 and SAP2 (Supplementary Fig. 2A, B ). To understand the evolutionary conservation of SAP1 and SAP2 protein sequences, we searched for SAP1 and SAP2 homologs in the Brassicaceae family, to which A. thaliana belongs, as well as in the more distant plant species, tomato and rice. All analyzed species have one to three SAP homologs (Supplementary Fig. 3A, B ), and expression of most of these genes was induced by flg22 (rice was not tested) (Supplementary Fig. 3C ), suggesting that the importance of SAPs in antibacterial defense is evolutionarily conserved. Seven Asp residues including one in the active site and the substituted Ser are conserved in all SAP homologs (Supplementary Fig. 2A and Fig. 3a ), pointing to the importance of these residues for SAP function. We produced recombinant SAP1 variants in which these eight amino acid residues were substituted with Ala and tested them for protease and in vitro bacterial suppression activity (Supplementary Fig. 2C-E ). Similar to the GFP control, D63A and D63/136A SAP1 variants showed no protease activity, although protein levels were similar to the other variants (Fig. 3c and Supplementary Fig. 2C, E ). Notably, these inactive variants did not suppress in vitro Pto growth (Fig. 3d and Supplementary Fig. 2D ), indicating that SAP1 protease activity is essential for its function in in vitro Pto growth suppression. Overexpression of the non-active variant SAP1 D63/136A in plants, which did not influence PR1 expression, plant growth, and reproduction (Fig. 2e–j ), had no effect on plant resistance against Pto (Fig. 2h ). Taken together, these results demonstrate that SAP1, annotated as a pseudopeptidase, functions as an active aspartic protease that suppresses Pto growth in vitro and in planta via its protease activity. Fig. 3 Secreted aspartic protease 1 (SAP1) and SAP2 cleave MucD. a , c Protease activity of purified GFP (green fluorescent protein), SAP1, SAP2 ( a ), and SAP1 D63/136A ( c ) protein. PepA, the aspartic protease inhibitor, pepstatin A. Data represent means and s.e.m of three biological replicates. Asterisks indicate significant differences (Student’s two-tailed t test; ** P < 0.01). b , d In vitro growth of Pto (OD 600 = 0.05) in minimal medium supplemented with purified recombinant proteins or boiled (b) recombinant proteins at 9 h after culturing. Data represent means and s.e.m. of four biological replicates. Asterisks indicate significant differences (Student’s two-tailed t ; * P < 0.05, ** P < 0.01). e Proteins extracted from bacterial culture medium incubated with SAP1, boiled SAP1 (SAP1(b)), or without SAP were visualized (Coomassie Brilliant Blue (CBB) staining). f MucD-His incubated with SAP1-GST, SAP1 D63/136A -GST, and SAP2-GST were visualized by immunoblotting using an anti-GST or anti-His antibody. Three independent experiments were performed with similar results. g , h Pto Δ mucD expressing MucD-HA (hemagglutinin) (OD 600 = 0.05) was infiltrated into leaves of 4-week-old Col, pUB::SAP1-RFP , and sap1 sap2 plants. MucD-HA in total protein at the indicated time points was detected by immunoblotting using an anti-HA antibody. CBB staining serves as protein loading control. Experiments were repeated at least three times with similar results Full size image SAP1 cleaves Pto MucD To elucidate how SAP1 suppresses Pto growth, in vitro bacterial culture was incubated with SAP1-GST or heat-inactivated SAP1-GST, and proteins from bacterial cells and the medium were separated by gel electrophoresis. Although there were no apparent differences in the band pattern of proteins from bacterial cells, we observed that the intensity of one band of a molecular weight of ~50 kDa in the medium was reduced specifically by incubation with the active SAP1-GST (Fig. 3e ). The corresponding protein band was subjected to liquid chromatography with tandem mass spectrometry (LC-MS/MS) analysis to identify SAP1-target Pto proteins (SAPTs). 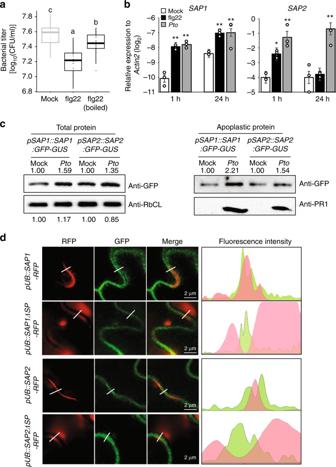Fig. 1 Secreted aspartic protease 1 (SAP1) and SAP2 are induced and secreted duringP. syringaeinfection.aIn vitro growth ofPto(OD600= 0.05) amended with apoplastic fluid from leaves of -week-old Col plants at 24 h post infiltration (hpi) with 1 µM flg22 or mock or boiled apoplastic fluid (boiled) was measured at 9 h after culturing. Bars represent means and s.e.m. of three independent experiments each with eight replicates. Statistically significant differences are indicated by different letters (adjustedP< 0.05).bExpression ofSAP1andSAP2in leaves of 4-week-old Col plants at 1 or 24 hpi with mock, 1 µM flg22, orPto(OD600= 0.001). Bars represent means and s.e.m. of three biological replicates. Asterisks indicate significant differences (Student’s two-tailedttest; *P< 0.05, **P< 0.01).cAccumulation of SAP1-GFP (green fluorescent protein) and SAP2-GFP at 1 day post infiltration (dpi) withPto(OD600= 0.001) or mock determined by immunoblotting using an anti-GFP antibody. Rubisco large subunit (RbCL) and PR1 serve as controls for total and apoplastic proteins, respectively.dSAP1-RFP (red fluorescent protein) and SAP2-RFP (red color) with or without the signal peptide (ΔSP) were expressed from the 35S promoter byAgrobacterium-mediated transient transformation in transgenicA. thalianaplants expressing plasma-membrane-localized WAVE131-YFP (yellow fluorescent protein) (green color). YFP and RFP fluorescence signals were detected at 2 dpi. The intensity of YFP and RFP fluorescence signals was quantified along the dotted lines using ImageJ software (left to right). Four independent experiments were performed with similar results Mapping of detected peptides to the Pto proteome resulted in 21 SAPT candidates with a reduced peptide levels in the active SAP1-GST sample (Supplementary Table 1 ). The top SAPT candidate containing a putative aspartic protease digestion site(s) was MucD, which is an HtrA-like protease involved in the regulation of alginate biosynthesis and in the responses to heat and oxidative stress [36] , [37] . A MucD homolog in the human opportunistic bacterial pathogen Pseudomonas aeruginosa is known to function as a serine protease and is important for virulence in animals as well as in plants [36] , [38] . An in vitro cleavage assay showed that SAP1 and SAP2 could cleave MucD, but that the protease-dead variant SAP1 D63/136A and the GFP control could not (Fig. 3f ). To investigate whether MucD cleavage occurs in planta, Pto expressing MucD-HA was infiltrated into leaves of Col plants, and MucD cleavage was monitored. The cleaved MucD product was detected in Col plants (Fig. 3g ). The detected bands were specific to MucD-HA as the bands were not detected using protein extracted from plants infected with wild-type Pto (Supplementary Fig. 4A ). MucD cleavage was enhanced in pUB::SAP1-RFP plants as compared to Col and pUB::SAP1 D63/136A -RFP plants (Fig. 3g and Supplementary Fig. 4B ). MucD cleavage was slightly reduced in single sap1 and sap2 mutant and sap1 SAP2-RNAi plants (Supplementary Fig. 4C, D ), and almost undetectable in sap1 sap2 CRISPR double mutant plants (Fig. 3h ). These results indicate that SAP1 and SAP2 are required to cleave Pto MucD during infection. The minor MucD cleavage detected in sap1 sap2 mutant plants suggests that SAP1 and SAP2 are the major enzymes that cleave Pto MucD, while other enzymes might also be involved in MucD cleavage. mucD is required for in planta Pto growth To determine whether mucD is important for Pto growth, mucD deletion mutants (Δ mucD ) and complemented lines (MucD-HA) of Pto were generated. Pto Δ mucD showed a mucoid phenotype probably due to overproduction of alginate [39] , and the complementation line exhibited a wild-type-like phenotype (Supplementary Fig. 5A ). We found that Pto MucD localized to the membrane, but was also secreted outside the cell (Supplementary Fig. 5B ) as in P. aeruginosa [38] , [39] . Compared to wild-type Pto , in vitro growth of Pto Δ mucD was slower and in planta growth was severely compromised, phenotypes that were both rescued by MucD-HA complementation (Fig. 4d–g and Supplementary Fig. 5C, D ). These results indicate that mucD is required for optimal Pto growth in vitro and in planta. Fig. 4 Secreted aspartic protease (SAP)-mediated cleavage of MucD suppresses Pto growth. a Schematic diagram of putative aspartic protease cleavage sites in MucD. The phenylalanine (F) and serine (S) residues were replaced with tyrosine (Y) and alanine (A), respectively. b MucD-His, MucD F106Y -His, and MucD S394A -His proteins were incubated with SAP1-GST. MucD-His or SAP1-GST was visualized by immunoblotting using an anti-HA or anti-GST antibody, respectively. Three independent experiments were performed with similar results. c Pto Δ mucD expressing MucD-HA and MucD F106Y -HA (OD 600 = 0.05) was infiltrated into leaves of 4-week-old Col, pUB::SAP1-RFP , and pUB::SAP1 D63/136A -RFP plants. MucD-HA was detected by immunoblotting at 6 hours post infection. Experiments were repeated at least three times with similar results. d In vitro growth of Pto , Pto Δ mucD , and Pto Δ mucD expressing MucD-HA, MucD F106Y -HA, or MucD S394A -HA (OD 600 = 0.005) over time. Data represent means and s.e.m. of three independent experiments each with three biological replicates. e In vitro growth of Pto (OD 600 = 0.05) supplied with purified recombinant proteins at 9 h after culturing. Data represent means and s.e.m. of three independent experiments with four biological replicates. f , g Pto , Pto Δ mucD , and Pto Δ mucD expressing MucD-HA or MucD F106Y -HA were infiltrated into leaves of 4-week-old Col, pUB::SAP1-RFP , pUB::SAP1 D63/136A -RFP , and sap1 sap2 plants, and bacterial titer was determined at 2 days post infection (dpi). Bars represent means and s.e.m. of three independent experiments with at least three biological replicates. d–g Statistically significant differences are indicated by different letters (adjusted P < 0.01) Full size image SAP1 and SAP2 suppress Pto growth via MucD cleavage Based on in silico analysis, the MucD protein sequence was predicted to harbor two putative aspartic protease cleavage sites [40] (Fig. 4a ). We generated MucD F106Y and MucD S394A with a mutation at each of the putative cleavage sites by aspartic proteases and produced His-tag-fused recombinant proteins at the C terminus. In the in vitro cleavage assay, we observed that SAP1-GST cleaves MucD S394A but not MucD F106Y (Fig. 4b ). This is congruent with the size of the cleaved MucD product in vitro and in planta (Figs. 3f–h , 4b, c ). To test whether this holds true in planta, we generated Δ mucD lines complemented with MucD F106Y . We inoculated Col, pUB::SAP1-RFP , and pUB::SAP1 D63/136A -RFP plants with wild-type Pto and Pto Δ mucD MucD F106Y and detected cleavage of wild-type MucD but not MucD F106Y (Fig. 4c ). These results indicate that F106 is the amino acid residue in MucD that is critical for cleavage by SAP1 in vitro and in planta. MucD F106Y -HA but not MucD S394A -HA complemented the mucoid phenotype and in vitro growth of Pto Δ mucD , indicating that MucD F106Y is functional (Fig. 4d and Supplementary Fig. 5A, C ). Then, we asked whether MucD cleavage is required for SAP-mediated growth suppression of Pto . First, we tested whether SAP1 suppresses Pto Δ mucD MucD F106Y growth in vitro. SAP1 but not SAP1 D63/136A and GFP control suppressed in vitro growth of wild-type Pto and Pto Δ mucD MucD (Fig. 4e ). However, SAP1 did not suppress Pto Δ mucD MucD F106Y growth, indicating that MucD cleavage is essential for SAP1-mediated growth suppression of Pto in vitro (Fig. 4e ). We then tested whether MucD cleavage is required for SAP1-mediated immunity in planta. We infiltrated leaves of Col, pUB::SAP1-RFP , pUB::SAP2-RFP , pUB::SAP1 ΔSP -RFP , pUB::SAP2 ΔSP -RFP , and pUB::SAP1 D63/136A -RFP plants with wild-type Pto , Pto Δ mucD , or Pto Δ mucD complemented with MucD-HA, MucD F106Y , or MucD S394A and determined in planta bacterial growth. As described above, Pto Δ mucD growth was compromised and was not different in different host plants (Fig. 4f, g and Supplementary Fig. 5D ). In planta growth of wild-type Pto and Pto Δ mucD MucD-HA was decreased only in plants overexpressing secreted and active SAP1 or SAP2 as compared with wild-type Col plants (Fig. 4f and Supplementary Fig. 5D ). Notably, growth of Pto Δ mucD MucD F106Y was not affected by SAP1 and SAP2 overexpression and was enhanced as compared to wild-type Pto , likely because Pto MucD F106Y could avoid SAP1- or SAP2-mediated cleavage (Fig. 4f and Supplementary Fig. 5D ). These results indicate that MucD cleavage was the cause of the enhanced resistance against Pto in SAP -overexpressing plants. To further demonstrate the physiological significance of SAP-mediated MucD cleavage, we infiltrated leaves of Col and sap1 sap2 CRISPR-knockout plants with wild-type Pto , Pto Δ mucD , or Pto Δ mucD complemented with MucD-HA or MucD F106Y -HA and determined in planta bacterial growth. As expected, the growth of wild-type Pto and Pto Δ mucD MucD-HA was enhanced in sap1 sap2 double mutant plants (Fig. 4g ). However, Pto Δ mucD MucD F106Y -HA growth was not affected by sap1 sap2 mutations (Fig. 4g ). Taken together, these results suggest that SAP1 and SAP2 cleave MucD, thereby suppressing Pto growth, and that MucD is the major bacterial target of SAP1 and SAP2 for plant immunity. A previous report showed that the activity of an aspartic protease, CDR1, triggers immune activation in A. thaliana [21] . As overexpression of SAP1 and SAP2 did not influence Pto Δ mucD MucD F106Y -HA growth in planta (Fig. 4f and Supplementary Fig. 5D ), activated immune response would be expected to be caused by MucD cleavage. Therefore, we tested whether cleaved fragments of MucD by SAP1 triggers activation of immune responses. We infiltrated leaves of Col plants with wild-type Pto or Pto Δ mucD MucD F106Y -HA and determined expression of the early immune marker gene FRK1 . To avoid differential immune activation by different bacterial populations, we collected samples at 6 h post infiltration (hpi), where in planta bacterial population of Pto and Pto Δ mucD MucD F106Y -HA were similar (Supplementary Fig. 5E ). We observed no significant difference in FRK1 expression levels between plants infiltrated with wild-type Pto or Pto Δ mucD MucD F106Y -HA (Supplementary Fig. 5F ). Thus, MucD cleavage by SAP1 and SAP2 unlikely triggers activation of an immune response effective for bacterial growth suppression. mucD exhibits site-specific diversity in Pseudomonas Comparative analysis of orthologous gene sequences retrieved from the KEGG database [41] ( n = 2304) indicates that MucD is highly conserved and widespread in bacteria (Fig. 5a ) but not in eukaryotes (Supplementary Data 1 ). This observation prompted us to test if SAP1 and SAP2 affect the growth of other microbial pathogens in plants. We found that SAP1 and SAP2 restricted the growth of Pseudomonas cannabina pv. alisalensis ES4326 ( Pca ES4326; formerly P. syringae pv. maculicola ES4326), in which MucD is identical to Pto MucD at the amino acid level, in a secretion-dependent manner, but did not affect the oomycete pathogen Albugo laibachii , which lacks MucD (Fig. 5d, e ). Thus, SAP1 and SAP2 may suppress growth of bacteria producing MucD, but have no effect on eukaryotes. Fig. 5 MucD is evolutionarily conserved. a Maximum-likelihood tree of MucD sequences ( n = 2304). Colors correspond to the different taxonomic groups. b Violin plots showing distributions of pairwise d N /d S ratios for each major taxonomic lineage as well as for the entire dataset. Sequences found in the genomes of Pseudomonas were removed from the “Gammaproteobacteria” and the “All” groups and were tested for significantly enriched d N /d S ratios (Mann–Whitney test; *** P < 0.001). c Distribution of site-variable d N /d S ratios for the multiple sequence alignment of mucD sequences found in Pseudomonas genomes ( n = 92). The color scale corresponds to the amino acid conservation rate at each site. Putative aspartic protease cleavage sites are indicated in red. d Pca E4326 (OD 600 = 0.001) was infiltrated into leaves of 4-week-old Col, pUB::SAP1-RFP and pUB::SAP2-RFP plants, and bacterial titer was determined at 2 dpi. Bars represent means and s.e.m of three independent experiments with three biological replicates. Asterisks indicate significant differences from Col (Student’s two-tailed t test; ** P < 0.01). e Col, pUB::SAP1-RFP , and pUB::SAP2-RFP were infected with Albugo laibachii , and the number of spores was measured at 14 dpi. Bars represent means and s.e.m. of three independent biological replicates Full size image Analysis of selection of bacterial mucD sequences using ratios of synonymous to non-synonymous mutations (d N /d S ) revealed strong signatures of purifying selection (Fig. 5b ). Interestingly, average d N /d S ratio across all sites were significantly higher in sequences from Pseudomonas genomes ( n = 92) compared to the rest of the dataset and to other Gammaproteobacteria ( n = 242; Fig. 5b ). Site-specific analysis of Pseudomonas orthologs revealed clusters of residues with higher d N /d S ratio that include F106 whose mutation blocks cleavage by SAP1 and SAP2 (Fig. 5c ), indicating that specific regions of mucD are under more positive selection in Pseudomonas . Positive selection (d N /d S > 1) is difficult to detect probably due to the high frequency of neutral and deleterious mutants. Thus, although d N /d S reaches only ~1, this result might suggest that plant SAPs impose selection pressure on bacterial mucD . During the Past three decades, a large amount of knowledge about how plants recognize microbial molecules and how signal is transduced within plant cells has been acquired. Nevertheless, it is still not understood how plant immunity suppresses the growth of bacterial pathogens that colonize in the apoplast. Here we show that the secreted plant proteases SAP1 and SAP2 serve as a front line of immunity, which inhibits bacterial growth. However, this cleavage of MucD by SAP1 and SAP2 does not appear to result in bacterial death as Pto Δ mucD is still viable. This mechanism of partial growth suppression, as opposed to total elimination of bacterial pathogens as is the case in animals [9] , [42] , might explain to some extent the finding that populations of non-virulent plant–bacterial pathogens do not decrease over time [43] . Furthermore, healthy plants in nature are surrounded by diverse bacterial communities that colonize the surface and interior of plant roots and leaves, which do not negatively impact plant fitness [43] , [44] , [45] , [46] , [47] . Our findings raise the possibility that secreted plant proteases such as SAP1 and SAP2 might contribute to shaping the plant microbiota and act as a gateway for control of non-virulent and commensal as well as pathogenic bacterial proliferation. It remains to be tested whether SAP-mediated suppression of bacterial growth also occurs in the case of plant endophytes containing MucD from other taxonomic groups and whether the increased positive selection observed in Pseudomonas corresponds to an adaptation against SAP-mediated MucD cleavage. Irrespective of this, our work identifies a molecular mechanism by which plant immunity suppresses growth of the bacterial pathogen Pto , likely in a direct manner. Over activation of immunity caused by intraspecific genetic incompatibilities, genetic engineering, or spontaneous mutations increases plant resistance against pathogens but often comes with a growth penalty [6] , [7] , [8] . This so-called immunity-growth tradeoff is shown to be genetically controlled in some cases, which makes production of highly resistant crops that retain growth a difficult task [48] , [49] . In contrast, overexpression of SAP in A. thaliana increases resistance against bacterial pathogens, but does not associate with growth retardation or reduced reproduction. Thus, boosting the direct targeting of pathogen factors by plant defense molecules may be an effective strategy to produce disease resistant crops without reducing yield. Our findings demonstrate that MucD cleavage is the cause of Pto growth suppression by SAP1 and SAP2 in A. thaliana . MucD from the human opportunistic pathogen P. aeruginosa localizes to the periplasm, the space between the inner cytoplasmic membrane and outer membrane, but is also secreted [37] , [38] . In a human cell line, P. aeruginosa MucD is secreted and cleaves interleukin-8, thereby suppressing host immunity [38] . Likewise, Pto MucD localizes to the membrane but is also secreted outside the cell. Thus, secreted Pto MucD may promote bacterial proliferation in plants and be cleaved by secreted SAP1 and SAP2 in the apoplast. Consistent with this, Pto harboring non-cleavable MucD shows higher virulence in plants compared with wild type. Alternatively, secreted SAP1 and SAP2 may also at least partly cleave MucD in the periplasm of Pto . Bacteria possess the ability to take up host proteins via membrane transporters [50] , [51] , [52] . Secreted SAP1 and SAP2 may exploit such systems to target MucD. In any case, our finding that both SAP and mucD are evolutionarily conserved in angiosperms and bacteria, respectively, provides an exciting avenue of research in plant–bacterial interactions. Plant materials and growth conditions Arabidopsis thaliana plants were grown in soil in a controlled environment at 22 °C with a 10 h light photoperiod and 65% relative humidity unless otherwise specified. For experiments in sterile conditions, seeds were sterilized with 1.5% sodium hypochlorite and 0.1% Triton X-100 and sown on half strength MS medium (containing half strength MS salts, including vitamins, 1% w/v sucrose, and 0.8% w/v plant agar, pH 5.8) in a controlled environment at 22 °C with a 10 h light photoperiod. All mutants and transgenic plants used in this study were in the background of the A. thaliana accession Col. T-DNA insertion lines for SAP1 (At1g03230; sap1-1 , SALK_062079 and sap1 -2, SAIL_646_E08) were obtained from the Nottingham Arabidopsis Stock Center. 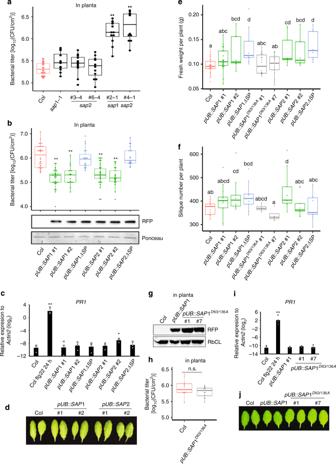Fig. 2 Secreted aspartic protease 1 (SAP1) andSAP2redundantly contribute to resistance againstP. syringae.aLeaves of 4-week-old Col,sap1,sap2, andsap1 sap2double mutant plants were infiltrated withPto(OD600= 0.0005), and bacterial titer was determined at 3 days post infection (dpi). Bars represent means and s.e.m. of four independent experiments with three biological replicates. Asterisks indicate significant differences from Col (Student’s two-tailedttest; *P< 0.05, **P< 0.01).bLeaves of 4-week-oldpUB::SAP1-RFP(red fluorescent protein) andSAP2-RFPwith or without signal peptide (ΔSP) were infiltrated withPto(OD600= 0.001), and bacterial titer was measured at 2 dpi. Bars represent means and s.e.m. of three independent experiments with at least three biological replicates. Asterisks indicate significant differences from Col (Student’s two-tailedttest; *P< 0.05, **P< 0.01). Protein expression determined by immunoblotting using an anti-RFP antibody. Ponceau S staining serves as protein loading control.c,iRelative expression ofPR1in leaves of 4-week-old Col,pUB::SAP1-RFP,pUB::SAP1ΔSP-RFP,pUB::SAP2-RFP,pUB::SAP2ΔSP-RFP, andpUB::SAP1D63/136Aplants were determined by quantitative reverse transcription PCR (RT-qPCR). Bars represent means and s.e.m of three biological replicates. The vertical axis shows the log2expression levels relative toActin2. Col plants 24 h post infiltration (hpi) with flg22 serves as a positive control for activatedPR1expression. Asterisks indicate significant differences from Col (Student’s two-tailedttest; *P< 0.05, **P< 0.01).d,jPhenotype of 4-week-old leaves of Col,pUB::SAP1-RFPandpUB::SAP2-RFP, andpUB::SAP1D63/136Aplants. Shoot fresh weight (4-week-old;e) and silique numbers (f) of Col,pUB::SAP1-RFP,pUB::SAP1ΔSP-RFP,pUB::SAP1D63/136A-RFP, pUB::SAP2-RFP, andpUB::SAP2ΔSP-RFPplants. Bars represent means and s.e.m. of three independent experiments each with four biological replicates (e) or means and s.e.m. of three independent experiments (f). Statistically significant differences are indicated by different letters (adjustedP< 0.01).gProtein expression of SAP1 and SAP1D63/136Ain Col,pUB::SAP1-RFPandpUB::SAP1D63/136A-RFPplants by immunoblotting using an anti-RFP antibody. Rubisco large subunit (RbCL) serves as a loading control. Three independent experiments were performed with similar results.hLeaves of 4-week-old Col andpUB::SAP1D63/136Aplants were infiltrated withPto(OD600= 0.001), and bacterial titer was measured at 2 dpi. Bars represent means and s.e.m, of four independent experiments with four biological replicates. n.s., not significant Homozygous T-DNA insertion mutants were verified by PCR using primers listed in Supplementary Table 2 . Accessions Capsella rubella (N22697) [53] , Arabidopsis lyrata (Mn47) [54] , Eutrema salsugineum (Shandong) [55] , and Solanum lycopersicum (Moneymaker) [56] were used. Transient expression in A. thaliana Agrobacterium tumefaciens -mediated transient transformation of A. thaliana seedlings was performed as described previously [57] . Briefly, A. tumefaciens was cultured in liquid YEB medium at 28 °C to OD 600 = 1.5, harvested by centrifugation, washed, and resuspended in 0.25× MS pH 6.0, 1% sucrose, 100 μM acetosyringone, and 0.005% Silwet L-77 to OD 600 = 0.5. The A. thaliana seedlings were co-cultivated with A. tumefaciens in a 96-well plate in the darkness for 36 h. GFP and RFP fluorescence was detected with an LSM700 confocal microscope (Zeiss Microscopy, Jena, Germany) at standard settings. Preparation of inocula and bacterial growth assay Pto strains [58] were grown overnight in King’s B medium supplemented with 50 µg/ml of rifampicin and P. cannabina pv. alisalensis ES4326 was grown overnight in King’s B medium supplemented with 50 µg/ml of streptomycin. The bacteria were harvested by centrifugation, washed, and diluted to the desired density with sterile water. The bacterial growth assay was performed as described before [59] . Briefly, 4- to 5-week old leaves were syringe inoculated with bacterial suspension using a needleless syringe. A leaf disc collected from the infiltrated leaf was considered a biological replicate. In each experiment, six different plants were infiltrated. RNA isolation and RT-qPCR Total RNA was isolated from plant samples using TRIzol reagent (Thermo Fisher Scientific) following the manufacturer’s instructions. Five micrograms of total RNA were reverse transcribed using the SuperScript II First-Strand Synthesis System (Thermo Fisher Scientific) with an oligo(dT) primer. Real-time DNA amplification was monitored using Bio-Rad iQ5 optical system software (Bio-Rad). The expression level of genes of interest was normalized to that of the endogenous reference gene ACTIN2 . The used primers are listed in Supplementary Table 2 . Extraction of apoplastic fluid Apoplastic fluid was extracted from 4-week-old A. thaliana leaves at 24 h post treatment with water or 1 µM of flg22. Leaves were collected and washed with sterilized water for two times. Leaves were submerged in sterilized water, vacuum infiltrated for 10 min, and released gently. Waters attached on leaves was carefully removed, and apoplastic fluid was collected after centrifuge at 1000 × g for 10 min at 4 °C. The extracted apoplastic fluid was filtered through a 0.22-µm filter. Total and apoplastic protein extraction Total and apoplastic protein was extracted from A. thaliana leaves as described previously [60] . Briefly, for total protein extraction, A. thaliana leaves were frozen in liquid nitrogen and ground to a fine powder. Protein extraction buffer (0.5 M Tris-HCl, pH 8.3, 2% v/v Nonidet P-40, 20 mM MgCl 2 , 2% v/v β-mercaptoethanol, 1 mM phenylmethylsulfonyl fluoride, and 1% w/v polyvinyl polypyrrolidine) and Tris-saturated phenol (pH 7.9) were added to the tissue powder, and then mixed gently at room temperature for 10 min. After centrifugation at 12,000 × g for 15 min at 4 °C, the phenol layer was transferred into a new tube and precipitated with methanol containing 100 mM ammonium acetate for 2 h at −20 °C. The precipitated protein pellet was washed twice with methanol containing 100 mM ammonium acetate and twice with 80% acetone. For apoplastic protein extraction, A. thaliana leaves were shaken in apoplastic extraction buffer (200 mM CaCl 2 , 5 mM sodium acetate pH 4.3, and protease inhibitor cocktail) on ice for 1 h. The extraction buffer was filtered through No. 2 filter paper (Whatman, Cambridge, UK) and mixed thoroughly after adding a half volume of Tris-saturated phenol. The phenolic phase was transferred into a new tube after centrifugation at 5000 × g for 15 min. Protein was precipitated and washed as described above. Immunoblotting Equal amounts of protein were separated by 12% sodium dodecyl sulfate-polyacrylamide gel electrophoresis (SDS-PAGE) and transferred to PVDF membranes (Sigma-Aldrich, St. Louis, MO, USA) with Mini-PROTEAN ® Tetra Handcast Systems (Bio-Rad, Hercules, CA, USA). The membranes were incubated with primary antibodies (for anti-GFP (Abcam, AB6556), 1:5000; anti-HA (Roche, 11867423001), 1:5000; anti-PR1, 1:5000; anti-RbCL (Clontech 632475), 1:2000; anti-GST (Virogen, 101-A-100), 1:5000; or anti-His (Thermo Fisher, PA1-23024), 1:5000) in 1× TBS with 5% w/v skim milk at 4 °C overnight. Treated membranes were washed with 1× TBS and incubated with a secondary horse radish peroxidase (HRP)-conjugated antibody (anti-rabbit HRP (Santa Cruz, sc-2004), 1:10,000; anti-rat (Santa Cruz, sc-2006), 1:10,000; anti-mouse (GE Healthcare Life Science; NA931), 1:10,000) at room temperature for 2 h. Signals were visualized using the Pierce ECL and ChemiDoc MP (Bio-Rad) systems. Protein band intensity was measured by using ImageJ software. Relative intensity protein band under Pto infection condition was calculated by normalizing to the intensity of protein band under mock condition, which was set as 1. Construction of transgenic plants The coding or promoter sequences of SAP1 (At1g03230) and SAP2 (At1g03220) were PCR amplified using the primers listed in Supplementary Table 2 , cloned into pENTR/D-TOPO (Thermo Fisher Scientific, Carlsbad, CA, USA), and transferred into pUB::C-RFP:GW or pFAST-G04 vectors [61] , respectively. To generate the SAP2 -RNAi line, a 547 bp fragment was amplified from the SAP2 coding sequence using the primers listed in Supplementary Table 2 , cloned into the pENTR/D-TOPO vector, and transferred into the pFAST-G03 vector [61] . Agrobacterium tumefaciens strain GV3101/pMP90 was transformed with each plasmid. The resultant agrobacteria were used to generate stable A. thaliana transgenic plants using the floral dip method (Clough and Bent, 1998). Transgenic plants were selected by spraying with BASTA (pUB::C-RFP:GW) or germinating on MS medium containing kanamycin (pFAST-G04) or hygromycin (pFAST-G03). The SAP2 CRISPR-CAS mutants were generated in Col and sap1-1 backgrounds with the CRISPR-Cas9 system from the Karlsruhe Institute of Technology following the provided protocol [62] , [63] , [64] . Identification of candidate SAP1 target proteins by LC-MS/MS Protein bands in silver-stained SDS-PAGE were excised with blades, washed with 50% v/v acetonitrile in 0.1 M NH 4 HCO 3 , and dried in a vacuum centrifuge. Gel fragments were treated with a reducing buffer (10 mM DTT, 0.1 M NH 4 HCO 3 ) for 45 min at 55 °C. After removal of the reducing buffer, 55 mM iodoacetamide in 0.1 M NH 4 HCO 3 was added. Gel pieces were then dried, submerged in digestion buffer (25 mM NH 4 HCO 3 , and 12.5 ng/ml trypsin), and incubated at 37 °C overnight. Tryptic peptides were analyzed by MS as previously described [65] . Recombinant protein expression and protease activity assay GFP , SAP1 , and site-mutagenized SAP1 and SAP2 were cloned into pDEST15 (Thermo Fisher Scientific), and mucD was cloned into pDEST59 (Invitrogen) for recombinant protein expression. The recombinant proteins were expressed in E. coli and purified through affinity pull-down with Pierce Glutathione agarose beads (Thermo Fisher Scientific) or Ni-NTA agarose beads (Qiagen, Hilden, Germany) according to the supplier’s instructions. The universal protease activity assay was carried out using purified recombinant protein as described previously [66] . Briefly, recombinant protein was added to a 0.65% w/v casein solution, and followed by incubation at 37 °C for 10 min. Trichloroacetic acid solution (110 mM) was added to stop the reaction, and the solution was incubated at 37 °C for 30 min. The supernatant was collected by filtration through a 0.45 µm polyethersulfone syringe filter. Folin and Ciocalteu’s phenol reagent (Sigma-Aldrich) and 500 mM sodium carbonate solution were added to the filtered solution (1:2 v/v and 2.5:1 v/v), respectively. The samples were then mixed and incubated at 37 °C for 30 min. The solution was collected after centrifugation at 3,000 × g for 10 min, and absorbance was measured by a spectrophotometer at 660 nm. Enzyme activity was calculated based on a standard curve using l -tyrosine as the standard. Pepstatin A (Sigma-Aldrich) was used as an aspartic protease inhibitor. Pepstatin A was pre-incubated with the purified recombinant protein at a concentration of 1 µM for 10 min prior to the protease activity assay. Generation of bacterial mutant and complementation lines A Pto mucD (PSPTO_4221) gene deletion mutant was created as previously described [67] . The upstream and downstream adjacent regions of mucD and a gentamycin resistance gene were amplified and linked together by PCR. This PCR product was then digested with Bam HI and Hin dIII and cloned into the MCS of pK18mobsacB [67] . The plasmid was then used to generate Δ mucD by a triparental mating using the helper plasmid pRK2013. The mucD coding sequence was amplified from Pto genomic DNA by PCR and cloned into the pENTR/D-TOPO vector, and then transferred to pCPP5040 by LR reaction. The complementation strains generated by a triparental mating of E. coli carrying pCPP5040::MucD-HA, pCPP5040::MucD F106Y -HA, or pCPP5040::MucD S394A -HA with the mucD deletion strain and a strain carrying pRK2013 and were selected with 50 µg/ml rifampicin, 5 µg/ml gentamycin, and 35 µg/ml chloramphenicol. Bacterial membrane and secreted protein extraction Pto MucD-HA was grown in King’s B medium overnight, washed with water twice, inoculated into M9 minimal medium (start OD 600 = 0.05), and cultured at 28 °C for 6 h. After centrifugation at 6000 × g for 10 min, bacterial cells and culture medium were used for membrane protein and secreted protein extraction, respectively. A carbonate extraction method was used for bacterial cell membrane isolation [68] . Briefly, the cell pellet was washed with wash solution (50 mM Tris-HCl, pH 7.5) and centrifuged at 2500 × g for 8 min. The pellet was then resuspended in wash solution containing DNase I. The cells were ruptured by sonication, and unbroken cells were removed by centrifugation at 2500 × g for 8 min. The supernatant was directly added to ice-cold 100 mM sodium carbonate solution, and gently stirred on ice for 1 h. The cell membranes were collected by ultracentrifugation at 115,000 × g for 1 h at 4 °C. The membrane pellet was resuspended in the wash solution, and collected by ultracentrifugation. Secreted protein in the culture medium was extracted with the phenol method [69] . Briefly, the culture medium was centrifuged again at 12,000 × g for 10 min, and the supernatant was collected and mixed with Tris-saturated phenol. After thorough mixing, the phenolic layer was collected by centrifugation at 3000 × g for 10 min. Protein was precipitated and washed as described above. Evolutionary analysis of bacterial mucD sequences We first retrieved all mucD -orthologous sequences found in the bacterial genomes present in the KEGG Ortholog (KO) database [41] (accessed on 15/10/2016). Next, we performed a multiple sequence alignment at the amino acid level using Clustal Omega [70] . Nucleotide sequences were then aligned by codon using Pal2Nal [71] . Based on this multiple sequence alignment, a species tree was inferred using FastTree [72] . We then employed the PAML software [73] to obtain, for each taxonomic group, pairwise d N /d S ratios using the M0 model and separately for sequences retrieved from Pseudomonas genomes using the M8 model, which allows d N /d S ratios to vary among sites. Distributions of pairwise d N /d S ratios were compared using the non-parametric Mann–Whitney test. P values were corrected for multiple testing using the Bonferroni method, with a significance threshold of α = 0.05. Albugo preparation and infection Albugo laibachii Nc14 spores from infected Col plants were collected from leaf washes and treated on ice for 30 min to release zoospores. Zoospores were collected by filtration and sprayed on A. thaliana leaves at a concentration of 5 × 10 4 conidiospores/ml. The inoculated plants were maintained in a growth chamber at 22 °C 16 h day/16 °C 8 h night with 100% relative humidity, and then moved to 75% relative humidity conditions after 36 h. The number of released spores on leaves were counted at 14 days post infiltration (dpi) as described previously [74] . Phylogenetic analysis of SAP1 homologs The entire protein sequences of A. thaliana , A. lyrata , C. rubella , C. grandiflora , E. salsugineum , B. rapa , tomato, and rice were retrieved from Phytozome [75] and used for identification of putative orthologous groups using the OrthoMCL program [76] . The used genes were CrubASP1 (Crubv10011636m), CrubASP2 (Crubv10025694m) AlyrASP1 (Alyr484681), AlyrASP2 (Alyr470302), EsalASP (Esalv10007672), SolycASP (Solyc01g080010.2.1), OsSAPa (Os05g33400.1), OsSAPb (Os05g33410.1), and OsSAPc (Os05g33430.1). The proteins belonging to the same group as A. thaliana SAP1 and SAP2 were aligned using MUSCLE [77] . A maximum likelihood phylogenetic tree was constructed using the MEGA6 software [78] . Statistical analysis The following models were fit to the relative cycle threshold (Ct) values compared to Actin2 (for qRT-PCR) or log 10 -transformed bacterial titers (for bacterial titer) with the lmer function in the lme4 package or the lm function in the R environment: C tgytr = GϒT gyt + R r + ɛ gytr , where GϒT is the genotype–treatment–time interaction, and random factors; R the biological replicate; ɛ the residual; C tgyr = Gϒ gy + R r + ɛ gytr , where Gϒ is the genotype–treatment interaction; C tgtr = GT gt + R r + ɛ gtr , where GT is the genotype–time interaction. The mean estimates of the fixed factors were used as the modeled relative Ct values visualized as the relative log 2 expression values or bacterial titers. Differences between estimated means were compared using two-tailed t tests. For the t tests, the standard errors appropriate for the comparisons were calculated with the variance and covariance values obtained from the model fittings. The Benjamini–Hochberg method was applied to correct for multiple hypothesis testing when all pairwise comparisons of the mean estimates were made. 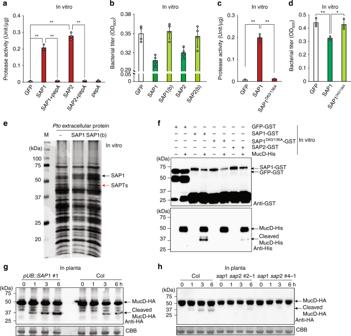Fig. 3 Secreted aspartic protease 1 (SAP1) and SAP2 cleave MucD.a,cProtease activity of purified GFP (green fluorescent protein), SAP1, SAP2 (a), and SAP1D63/136A(c) protein. PepA, the aspartic protease inhibitor, pepstatin A. Data represent means and s.e.m of three biological replicates. Asterisks indicate significant differences (Student’s two-tailedttest; **P< 0.01).b,dIn vitro growth ofPto(OD600= 0.05) in minimal medium supplemented with purified recombinant proteins or boiled (b) recombinant proteins at 9 h after culturing. Data represent means and s.e.m. of four biological replicates. Asterisks indicate significant differences (Student’s two-tailedt; *P< 0.05, **P< 0.01).eProteins extracted from bacterial culture medium incubated with SAP1, boiled SAP1 (SAP1(b)), or without SAP were visualized (Coomassie Brilliant Blue (CBB) staining).fMucD-His incubated with SAP1-GST, SAP1D63/136A-GST, and SAP2-GST were visualized by immunoblotting using an anti-GST or anti-His antibody. Three independent experiments were performed with similar results.g,hPtoΔmucDexpressing MucD-HA (hemagglutinin) (OD600= 0.05) was infiltrated into leaves of 4-week-old Col,pUB::SAP1-RFP, andsap1 sap2plants. MucD-HA in total protein at the indicated time points was detected by immunoblotting using an anti-HA antibody. CBB staining serves as protein loading control. Experiments were repeated at least three times with similar results 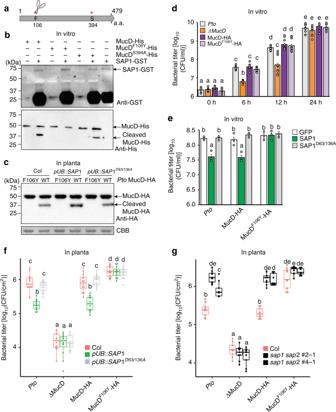Fig. 4 Secreted aspartic protease (SAP)-mediated cleavage of MucD suppressesPtogrowth.aSchematic diagram of putative aspartic protease cleavage sites in MucD. The phenylalanine (F) and serine (S) residues were replaced with tyrosine (Y) and alanine (A), respectively.bMucD-His, MucDF106Y-His, and MucDS394A-His proteins were incubated with SAP1-GST. MucD-His or SAP1-GST was visualized by immunoblotting using an anti-HA or anti-GST antibody, respectively. Three independent experiments were performed with similar results.cPtoΔmucDexpressing MucD-HA and MucDF106Y-HA (OD600= 0.05) was infiltrated into leaves of 4-week-old Col,pUB::SAP1-RFP, andpUB::SAP1D63/136A-RFPplants. MucD-HA was detected by immunoblotting at 6 hours post infection. Experiments were repeated at least three times with similar results.dIn vitro growth ofPto,PtoΔmucD, andPtoΔmucDexpressing MucD-HA, MucDF106Y-HA, or MucDS394A-HA (OD600= 0.005) over time. Data represent means and s.e.m. of three independent experiments each with three biological replicates.eIn vitro growth ofPto(OD600= 0.05) supplied with purified recombinant proteins at 9 h after culturing. Data represent means and s.e.m. of three independent experiments with four biological replicates.f,gPto,PtoΔmucD, andPtoΔmucDexpressing MucD-HA or MucDF106Y-HA were infiltrated into leaves of 4-week-old Col,pUB::SAP1-RFP,pUB::SAP1D63/136A-RFP, andsap1 sap2plants, and bacterial titer was determined at 2 days post infection (dpi). Bars represent means and s.e.m. of three independent experiments with at least three biological replicates.d–gStatistically significant differences are indicated by different letters (adjustedP< 0.01) 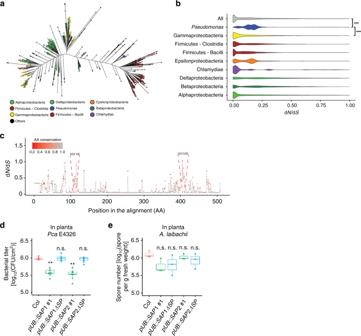Fig. 5 MucD is evolutionarily conserved.aMaximum-likelihood tree of MucD sequences (n= 2304). Colors correspond to the different taxonomic groups.bViolin plots showing distributions of pairwise dN/dSratios for each major taxonomic lineage as well as for the entire dataset. Sequences found in the genomes ofPseudomonaswere removed from the “Gammaproteobacteria” and the “All” groups and were tested for significantly enriched dN/dSratios (Mann–Whitney test; ***P< 0.001).cDistribution of site-variable dN/dSratios for the multiple sequence alignment of mucD sequences found inPseudomonasgenomes (n= 92). The color scale corresponds to the amino acid conservation rate at each site. Putative aspartic protease cleavage sites are indicated in red.dPcaE4326 (OD600= 0.001) was infiltrated into leaves of 4-week-old Col,pUB::SAP1-RFPandpUB::SAP2-RFPplants, and bacterial titer was determined at 2 dpi. Bars represent means and s.e.m of three independent experiments with three biological replicates. Asterisks indicate significant differences from Col (Student’s two-tailedttest; **P< 0.01).eCol,pUB::SAP1-RFP, andpUB::SAP2-RFPwere infected withAlbugo laibachii, and the number of spores was measured at 14 dpi. Bars represent means and s.e.m. of three independent biological replicates Reporting summary Further information on research design is available in the Nature Research Reporting Summary linked to this article.